Metabolic enzyme expression highlights a key role for MTHFD2 and the mitochondrial folate pathway in cancer Metabolic remodeling is now widely regarded as a hallmark of cancer, but it is not clear whether individual metabolic strategies are frequently exploited by many tumours. Here we compare messenger RNA profiles of 1,454 metabolic enzymes across 1,981 tumours spanning 19 cancer types to identify enzymes that are consistently differentially expressed. Our meta-analysis recovers established targets of some of the most widely used chemotherapeutics, including dihydrofolate reductase, thymidylate synthase and ribonucleotide reductase, while also spotlighting new enzymes, such as the mitochondrial proline biosynthetic enzyme PYCR1 . The highest scoring pathway is mitochondrial one-carbon metabolism and is centred on MTHFD2 . MTHFD2 RNA and protein are markedly elevated in many cancers and correlated with poor survival in breast cancer. MTHFD2 is expressed in the developing embryo, but is absent in most healthy adult tissues, even those that are proliferating. Our study highlights the importance of mitochondrial compartmentalization of one-carbon metabolism in cancer and raises important therapeutic hypotheses. Divergent metabolism in tumours was first recognized nearly a century ago [1] , is consistently observed across a number of tumour types, and has been exploited for diagnostic as well as therapeutic purposes. For example, rapid glucose consumption in tumours may be imaged by positron emission tomography and used to diagnose malignancy and to monitor the response to therapy [2] . Furthermore, the dependence of cancer cells on nucleotide metabolism forms the basis for the use of several common chemotherapeutics, including agents targeting dihydrofolate reductase (DHFR), thymidylate synthase (TYMS) and ribonucleotide reductase (RRM2) [3] . Moreover, recent data have suggested that many of the growth factor signalling pathways commonly perturbed in cancer impinge on metabolic enzymes [4] , as well as that metabolic enzymes may act as bona fide oncogenes [5] and even transform cells [6] . Collectively, these observations underscore the need for a deeper understanding of metabolic reprogramming in cancer. While classic biochemical studies have identified a number of enzymes whose activities are increased in cancers [7] , [8] , the complex, coordinated changes in metabolism that occur during cancer transformation have only begun to be understood [9] . Over the past decade, a wealth of data on tumours, normal tissues and cell models have been generated using microarrays and analysed to identify genes differentially expressed in cancer [10] , [11] . These data provide a unique opportunity to study expression patterns of metabolic enzymes in cancer and thereby define the metabolic programme of cancer on a genome-wide scale [9] . Yet, as most studies have compared tumour tissue with a quiescent, postmitotic normal control tissue, these analyses do not indicate whether enzymes overexpressed in tumours are also active in proliferative normal tissues. Identification of cancer-specific metabolic activities is essential, as current chemotherapeutic agents target metabolic enzymes found both in transformed cells as well as normal proliferating cells, notably immune cells, hair follicles and intestinal epithelium, resulting in the on-target side effects in proliferative tissues that limit these agents’ therapeutic index [3] . Here we report a systematic re-analysis of previously published microarray data sets, focusing on genes known or predicted to encode metabolic enzymes, and identify several enzymes and pathways consistently overexpressed or underexpressed across a large number of different cancer types. In particular, we find that enzymes of the mitochondrial folate metabolic pathway, which are ordinarily low or absent in normal adult tissues, are highly upregulated in cancer. Finally, we show that the MTHFD2 enzyme in this pathway is highly expressed on the protein level in a variety of human tumours and negatively correlates with survival in breast cancer patients. Meta-analysis of enzyme mRNA expression in human tumours To systematically investigate expression of metabolic pathways across multiple tumour types, we first searched the GeneChip Oncology Database (GCOD) [10] for studies containing primary tumour tissue samples and suitable normal tissue controls. We found 51 independent data sets satisfying this criterion, covering a total of 1,981 tumours of 19 different types versus 931 matched normal tissue controls ( Supplementary Data 1 ), and interrogating a total of 20,103 genes. To avoid artifacts from comparison across different array platforms and laboratories, we calculated the differential expression (quantified by Z -scores) within each data set and estimated the statistical significance for each gene by permutation tests. While the extent of differential expression varied widely across studies ( Fig. 1a )—likely reflecting variability in tumour types, nature of the control tissue and experimental design—we reasoned that genes consistently differentially expressed across these cancers would represent processes of fundamental importance to transformed cells. We therefore scored each gene by counting the number of data sets where differential expression was detected at a 5% false discovery rate (FDR) ( Fig. 1b , full genome-wide analysis available as Supplementary Data 2 ). Most high-scoring overexpressed genes have previously been found to be expressed in the ‘committed’ S, G2 and M phases of the cell cycle [12] , [13] , where cells are thought to be most vulnerable to pharmacologic intervention. This likely reflects the high proportion of proliferating cells in tumours compared with control tissues. 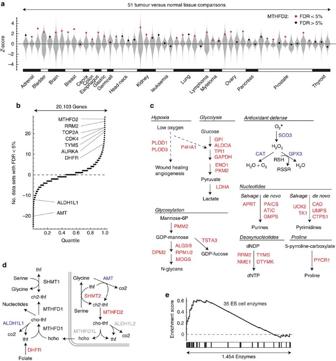Figure 1: Transcriptional regulation of metabolic pathways in human tumours. (a) Differential expression (Z-score) distributions for 51 tumour-versus-normal data sets representing 19 tumour types are shown as violin plots (grey). Dots indicateZ-scores forMTHFD2in each study; red colour denotes significance at <5% FDR. (b) Distribution of meta-analysis scores for all 20,103 genes interrogated across the 51 data sets. Gene symbols indicated, see text for further description. (c) Metabolic pathways detected as strongly overexpressed (among top 50 metabolic enzymes; red gene symbols) or underexpressed (among bottom 50 metabolic enzymes; blue gene symbols) in tumours. (d) Schematic of one-carbon metabolism with overexpressed (red) and underexpressed (blue) genes indicated. Grey symbols, not measured. (e) Gene set enrichment analysis for the set of 35 embryonic metabolic enzymes compared with mRNAs for all enzymes. Figure 1: Transcriptional regulation of metabolic pathways in human tumours. ( a ) Differential expression ( Z -score) distributions for 51 tumour-versus-normal data sets representing 19 tumour types are shown as violin plots (grey). Dots indicate Z -scores for MTHFD2 in each study; red colour denotes significance at <5% FDR. ( b ) Distribution of meta-analysis scores for all 20,103 genes interrogated across the 51 data sets. Gene symbols indicated, see text for further description. ( c ) Metabolic pathways detected as strongly overexpressed (among top 50 metabolic enzymes; red gene symbols) or underexpressed (among bottom 50 metabolic enzymes; blue gene symbols) in tumours. ( d ) Schematic of one-carbon metabolism with overexpressed (red) and underexpressed (blue) genes indicated. Grey symbols, not measured. ( e ) Gene set enrichment analysis for the set of 35 embryonic metabolic enzymes compared with mRNAs for all enzymes. Full size image We focused our analysis on 1,454 metabolic enzymes annotated in a previously established model of the human metabolic network [14] . Among the top 50 consistently overexpressed enzymes ( Table 1 ), we recovered several metabolic pathways previously associated with cancer, including multiple enzymes involved in glycolysis [15] , de novo synthesis and salvage of nucleotides [7] and in particular deoxynucleotides, as well as prolyl hydroxylases responsive to hypoxia [16] and glycosylation enzymes [17] ( Fig. 1c,d ), in agreement with a recent independent study [9] . Among these metabolic enzymes, we recovered a number of genes targeted by existing cancer therapeutics, including DHFR (target of methotrexate), TYMS (target of 5-fluorouracil) and RRM2 (target of gemcitabine) ( Fig. 1b ; Table 1 ). Beyond metabolic enzymes, our analysis also identified a number of other enzymes targeted by chemotherapeutics, including topoisomerase 2A, aurora A kinase and cyclin-dependent kinase 4 ( Fig. 1b ; Supplementary Data 2 ), as consistently overexpressed in cancers. Hence, our systematic analysis of metabolic reprogramming identifies a number of established cancer-related metabolic enzymes and pathways across varied tumour types. Table 1 Top 50 metabolic enzymes frequently overexpressed in human tumours. Full size table Our analysis additionally reveals several metabolic enzymes consistently underexpressed in cancer and whose roles in cancer have not been previously appreciated. 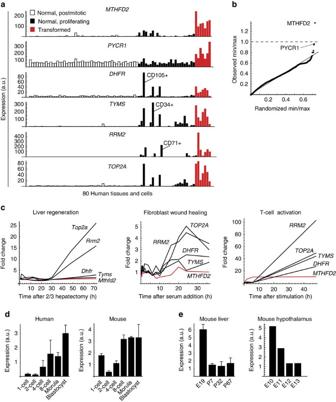Figure 2: MTHFD2 expression in transformed proliferating cells compared with normal proliferating cells. (a) mRNA expression levels in normal post-mitotic (open bars), normal proliferating (black bars) and transformed (red bars) cells or tissues forMTHFD2and four established cancer drug targets. Normal hematopoietic cell fractions with strong expression are indicated. (b) Quantile–quantile plot for the ratio of minimal expression among transformed cells to maximum expression among normal (proliferating and post-mitotic) cells, defined as in (a), for each of the 12,529 human mRNAs measured. Randomized quantiles (X-axis) were obtained by permuting samples.MTHFD2mRNA is indicated. (c) mRNA expression of humanMTHFD2or mouseMthfd2and four established cancer drug targets during mouse liver regeneration following partial hepatectomy (left); human fibroblasts proliferating in response to serum stimulation (center); and human CD4+ T lymphocytes activated by CD3 and CD28 antibodies (right). Red line indicatesMthfd2/MTHFD2. (d) mRNA expression of humanMTHFD2(left) and mouseMthfd2(right) during early embryonic development. Error bars denote s.d. (n=3). (e) mRNA expression of mouseMthfd2during embryonic development of liver (left) and hypothalamus (right). Error bars denote s.d. (n=2). Among the metabolic enzymes consistently underexpressed in cancer ( Table 2 ), we noted a number of enzymes related to fatty acid metabolism, including catabolism of branched fatty acids ( ACOX2 , ETFDH ), synthesis of ketones ( HMGCS2 ) and fatty acid synthesis ( ACACB ). A number of antioxidant enzymes were also consistently downregulated in cancer ( Fig. 1c ; Table 2 ). Taken together, these findings suggest consistent downregulated metabolic pathways and enzymes across multiple tumour types, which remain to be explored. Table 2 Top 50 metabolic enzymes frequently underexpressed in human tumours. Full size table Cancer cells have previously been proposed to exhibit stem cell-like properties, expressing genes characteristically found in embryonic cells [18] . Of the 35 enzymes previously established to be expressed by embryonic stem cells [18] , a large fraction were overexpressed in tumours ( Fig. 1e ), suggesting a tendency to revert to an embryonic-like metabolic programme. Among the top 50 consistently overexpressed enzymes ( Table 1 ) identified in our study, 26 enzymes have previously been evaluated using large-scale RNA interference (RNAi) screening to determine those essential for tumorgenesis in vitro and in vivo in breast cancer cells [19] . Among these 26 metabolic genes, six genes ( CTPS , GAPDH , PYCR1 , MTHFD2 , TPI1 and TSTA3 ) were found to be required for tumorgenesis in vitro and five genes ( CTPS , GAPDH , GMPS , PYCR1 and TPI1 ) in vivo [19] . Whereas several of these genes are components of glycolytic or nucleotide metabolism pathways previously associated with tumorgenesis; TSTA3 , PYCR1 and MTHFD2 are members of pathways less appreciated in the context of cancer. TSTA3 catalyses the production of GDP- L -fucose ( Fig. 1c ), which serves as the substrate for fucosyltransferases. Increased levels of GDP- L -fucose and fucosylated glycoproteins have been noted in cancer [20] ; their role in tumorgenesis remains unclear. Similarly, our analysis also identified the mitochondrial enzyme PYCR1 ( Fig. 1c ), an established target of the oncogene myc [21] . PYCR1 catalyses the final step of proline synthesis from glutamate ( Fig. 1c ), including in cancer cells [22] . In conjunction with its cytosolic isoform, PYCR1 may serve as a cycle for the transfer of reducing equivalents from the cytosol into the mitochondrion [23] , modulating both intracellular redox status [24] and sensitivity to oxidant injury [25] . Among all 1,454 enzymes examined, the metabolic enzyme most consistently overexpressed in tumours was the mitochondrial folate-coupled dehydrogenase MTHFD2 ( Fig. 1a,b ), ranked within the top three of all 20,103 genes interrogated ( Supplementary Data 2 ). MTHFD2 is integral to mitochondrial one-carbon metabolism ( Fig. 1d ), a metabolic system recently implicated in rapid cancer cell proliferation [26] . MTHFD2 is a bifunctional enzyme, catalysing the NAD + -dependent CH 2 -THF dehydrogenase and CH + -THF cyclohydrolase reactions within the mitochondria [27] . Within the mitochondrial one-carbon metabolism, we also noted frequent overexpression of the preceding enzyme, SHMT2 , which catalyses the production of glycine and one-carbon groups in the form of CH 2 -THF from serine ( Fig. 1d ). The subsequent enzyme, MTHFD1L , catalysing the synthesis of formate and regeneration of the THF cofactor ( Fig. 1d ), was only measured on 11/51 data sets, and our meta-analysis was not well-powered in this case; however, it appeared consistently overexpressed in those 11 data sets (data not shown). In the paralogous cytosolic one-carbon pathway, the NADP + -linked, trifunctional MTHFD1 enzyme also exhibited overexpression in multiple cancers, although it did not reach the top 50 threshold ( Fig. 1d ). This is consistent with the notion that the mitochondrial one-carbon system serves to produce formate that is then coupled to THF in the cytosol by the MTHFD1 enzyme [27] . Interestingly, the cytosolic enzyme ALDH1L1 , which breaks down cytosolic formyl-THF into CO 2 and THF and thus opposes the synthesis of one-carbon units, was consistently underexpressed in tumours ( Fig. 1d ; Table 2 ). The paralogous mitochondrial enzyme, ALDH1L2 was not reliably measured on the microarray platforms used ( Fig. 1d ). The aminomethyltransferase AMT , a component of the enzyme system that catabolizes glycine, was also underexpressed ( Fig. 1d ; Table 2 ). These findings suggest that the metabolic pathway channelling one-carbon units through the mitochondria via MTHFD2 has an important role in cancer biology. Enzymes in transformed and normal proliferating cells Many of the metabolic changes accompanying transformation are also active in normal proliferating cells [4] . To identify cancer-related metabolic enzymes more specific to the transformed state, we analysed gene expression from 80 normal human tissues, including proliferative tissues such as intestine and bone marrow, compared with transformed cell lines. The well-known chemotherapeutic targets DHFR , RRM2 , TYMS and topoisomerase 2A (TOP2A) were expressed in several normal proliferating cell types ( Fig. 2a ), in which the adverse side effects of drugs targeting these enzymes are commonly observed. In contrast, MTHFD2 exhibited little expression in these tissues, and was in fact the most cancer-specific messenger RNA (mRNA) measured on these arrays, as quantified by a transformed/normal expression ratio ( Fig. 2b ). In this analysis, we also noted the PYCR1 enzyme ( Fig. 2b ), which was also among the most commonly overexpressed enzymes in cancer ( Table 1 ). MTHFD2 was not detected in serum-stimulated normal human fibroblasts in vitro or in hepatocytes proliferating in vivo in response to partial liver resection ( Fig. 2c ), whereas other established chemotherapeutic drug targets were induced in these normal proliferating cells. However, we did observe MTHFD2 induction at an early time point in activated lymphocytes ( Fig. 2c ), consistent with previously observed MTHFD2 activity in bone marrow [28] , indicating a possible role for MTHFD2 in normal hematopoietic cells. Figure 2: MTHFD2 expression in transformed proliferating cells compared with normal proliferating cells. ( a ) mRNA expression levels in normal post-mitotic (open bars), normal proliferating (black bars) and transformed (red bars) cells or tissues for MTHFD2 and four established cancer drug targets. Normal hematopoietic cell fractions with strong expression are indicated. ( b ) Quantile–quantile plot for the ratio of minimal expression among transformed cells to maximum expression among normal (proliferating and post-mitotic) cells, defined as in ( a ), for each of the 12,529 human mRNAs measured. Randomized quantiles ( X -axis) were obtained by permuting samples. MTHFD2 mRNA is indicated. ( c ) mRNA expression of human MTHFD2 or mouse Mthfd2 and four established cancer drug targets during mouse liver regeneration following partial hepatectomy (left); human fibroblasts proliferating in response to serum stimulation (center); and human CD4+ T lymphocytes activated by CD3 and CD28 antibodies (right). Red line indicates Mthfd2 / MTHFD2 . ( d ) mRNA expression of human MTHFD2 (left) and mouse Mthfd2 (right) during early embryonic development. Error bars denote s.d. ( n =3). ( e ) mRNA expression of mouse Mthfd2 during embryonic development of liver (left) and hypothalamus (right). Error bars denote s.d. ( n =2). Full size image MTHFD2 enzymatic activity has previously been detected in mouse embryonic fibroblasts [28] as well as in human embryonic stem cells [18] , and Mthfd2 deletion is embyronic lethal in mice [29] . We found that the MTHFD2 mRNA increases during the initial rounds of cellular division in both mouse and human fertilized oocytes ( Fig. 2d ). In addition, expression is high in mouse fetal liver and hypothalamus, but decreases markedly around birth ( Fig. 2e ). These observations support a role for the enzyme in embryonic development. RNA interference targeting MTHFD2 causes cancer cell death To further evaluate whether expression of the MTHFD2 gene product is required for cancer cell proliferation, we used two different RNAi modalities to silence MTHFD2 across 16 diverse cancer cell types. In total, we used two lentiviral-delivered short hairpin RNAs (shRNAs) and six sequence-independent non-viral-delivered short interfering RNA (siRNA) oligonucleotides ( Supplementary Figs 1,2 ). MTHFD2 mRNA, protein levels and enzymatic activity were substantially reduced by shRNA ( Supplementary Figs 1a–c and 3 ) or siRNA targeting MTHFD2 ( Supplementary Fig. 1e ). In most cell lines, proliferation was severely reduced, consistent with prior observations [19] , with noted variability in the degree of defect among the various cell lines ( Supplementary Fig. 1d,f ). Propidium iodide (PI) staining and flow cytometry revealed marked cell death at the 48 h time point, with 40% of cells nonviable ( Supplementary Fig. 1g,h ), while non-targeting control siRNA transfections did not impair cell viability ( Supplementary Fig. 1i ). While RNAi-mediated loss of the MTHFD2 gene product was associated with slowed cancer cell proliferation and marked cell death, we have hitherto been unable to rescue this phenotype by exogenous expression of the MTHFD2 cDNA, which is required to definitively prove that the effect is due to the enzymatic activity of MTHFD2 protein and not a consequence of silencing its RNA or an off-target effect. MTHFD2 protein expression in tumours and normal tissues To evaluate whether the MTHFD2 protein is overexpressed in human tumours, we performed immunohistochemistry in 176 tumour samples, collected from 16 tumour types. Strong or moderate staining for MTHFD2 was observed in 12 of these tumour types, and the protein was detected in all cancer types with the exception of gliomas ( Fig. 3a ). While staining intensity was variable across tumour samples, the protein consistently appeared specific to transformed cells within the tumours, with little or no staining seen in adjacent stroma ( Fig. 3b ). These data indicate that the MTHFD2 protein is indeed present in multiple cancer types. Activity of the enzyme has also previously been observed in transformed cell lines [30] . We did observe staining in normal epithelium of the gut tissues, in particular in intestinal crypts containing stem cells, in tonsil lymphoid tissue and in exocrine pancreas ( Supplementary Fig. 4 ). Finally, we evaluated the expression of MTHFD2 in six independent cohorts of patients with breast cancer followed for survival. Whereas there was heterogeneity among individual data sets ( Supplementary Fig. 5a ), likely reflecting differences in the number of patients and clinical parameters including, entry patient criteria and treatment strategies, a meta-analysis of all six independent cohorts indicated that high expression of the MTHFD2 mRNA was associated with increased mortality in breast cancer patients ( Supplementary Fig. 5b ), suggesting a potential role in tumour progression. 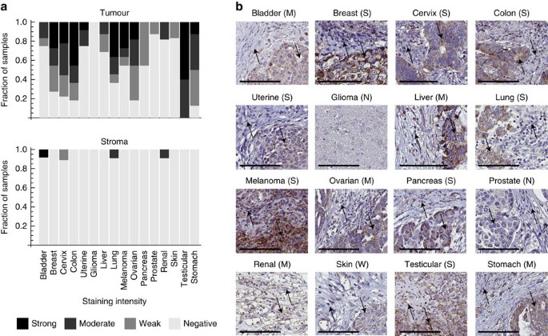Figure 3: MTHFD2 protein expression in human tumours. (a) Top, fraction of samples with none, weak, moderate or strong immunohistochemistry staining for MTHFD2 in transformed cells, across 16 solid tumour types. Bottom, same analysis as above for stromal cells. For each tumour type, tumours from nine to 12 individuals were examined. (b) Representative images from each of the 16 tumour types summarized in (a), exemplifying negative (N), weak (W), moderate (M) or strong (S) staining intensities. Up arrow, stromal cells; down arrow, cancer cells. Scale bar represent 100 μm. Figure 3: MTHFD2 protein expression in human tumours. ( a ) Top, fraction of samples with none, weak, moderate or strong immunohistochemistry staining for MTHFD2 in transformed cells, across 16 solid tumour types. Bottom, same analysis as above for stromal cells. For each tumour type, tumours from nine to 12 individuals were examined. ( b ) Representative images from each of the 16 tumour types summarized in ( a ), exemplifying negative (N), weak (W), moderate (M) or strong (S) staining intensities. Up arrow, stromal cells; down arrow, cancer cells. Scale bar represent 100 μm. Full size image In this study, we have identified metabolic enzymes and pathways that are frequently overexpressed in tumours, and demonstrated that one of these enzymes, MTHFD2 , is broadly required for cancer cell proliferation and viability. It should be emphasized that our meta-analysis only addresses changes in enzyme expression at the mRNA level, and our results do not exclude that other enzymes may be dysregulated in cancer by post-transcriptional mechanisms such as translational control or allosteric regulation. Moreover, while our meta-analysis was designed to reliably detect genes that are frequently overexpressed in tumours, it will likely miss genes absent or not well measured on common microarray platforms, and does not consider tissue-specific phenomena. Future studies investigating differences in metabolic enzyme expression between tumour types, as well as co-occurrence of enzymes and pathways in tumours, would be a valuable extension to this work. Within our systematic analysis of metabolic reprogramming, we identified a number of metabolic genes whose expression was altered in a variety of tumour types relative to normal controls. Among the metabolic enzymes that were consistently overexpressed in tumours ( Table 1 ), we find a high proportion of established cancer-related metabolic enzymes and known chemotherapeutic drug targets, suggesting that the additional enzymes identified here may be of interest as cancer targets as well. These additional enzymes include MTHFD2 and PYCR1 , both of which are low or absent in a large panel of normal tissues, including the proliferative tissues of the gut and a number of immune cell types; this could theoretically limit on-target side effects typically associated with these cell types. We further demonstrate the necessity of the MTHFD2 gene in cancer cell proliferation and survival across a number of cancer cell lines. While the proliferation defect and early cell death phenotypes with MTHFD2 knockdown were observed with multiple independent RNAi sequences, we cannot definitively rule out off-target RNAi effects. Moreover, while our results indicate a requirement for the MTHFD2 mRNA, further studies are needed to prove that the MTHFD2 protein and its enzymatic activity are indeed mediating the observed effects on cancer cell proliferation. Genes consistently underexpressed in tumours include metabolic enzymes involved in fatty acid metabolism, including catabolism of branched fatty acids and ketogenesis as well as a number of antioxidant enzymes ( Table 2 ). The consistent repression of these metabolic enzymes suggests a larger metabolic reprogramming that occurs with transformation in varied tumour types, and may reflect an effort on the part of a cancer cell to shunt metabolites to particular biosynthetic pathways rather than catabolism, to limit the production of toxic intermediates and/or to preferentially shuttle reducing equivalents to particular compartments, such as the mitochondria. As with the overexpressed metabolic genes, further investigation of these underexpressed metabolic enzymes may uncover metabolic vulnerabilities, which may be targeted therapeutically. While the enzymatic function of the MTHFD2 enzyme is well established, its broader role in cancer cell metabolism is not yet clear. Interestingly, while SHMT2 knockdown renders cancer cells auxotrophic for glycine [26] , we find that MTHFD2 knockdown results in death of human cancer cells in a complete medium containing glycine ( Supplementary Fig. 1g,h ). This observation indicates that the observed cell death on loss of MTHFD2 is not due to blocking of glycine synthesis. Moreover, as SHMT2 is thought to be the main source of mitochondrial one-carbon units, this observation also suggests that depletion of formate, the other main metabolic product of the mitochondrial one-carbon pathway, is unlikely to be the cause of cell death on loss of MTHFD2. In support of this hypothesis, we have been unable to rescue the MTHFD2 defect with exogenous formate. Moreover, both normal and transformed mouse embryonic fibroblasts lacking MTHFD2 are viable but auxotrophic for glycine [31] , suggesting that the strict dependence on MTHFD2 may be unique to human cells. A recent report indicates that RNAi targeting MTHFD2 also affects cell migration and invasion of human cancer cells [32] . The cell death observed on MTHFD2 depletion may therefore be due to some type of toxic event that does not arise in wild-type cells and is unrelated to normal cellular metabolism. One hypothesis is that, since MTHFD2 is considered required for recycling the THF cofactor in mitochondria ( Fig. 1d ), loss of the protein could result in mitochondrial folates becoming ‘trapped’ in the CH 2 -THF form, which would be detrimental to all folate-coupled activities in the mitochondria. In addition, because CH 2 -THF cannot be transported out of the mitochondria [27] , folate trapping within the mitochondria with MTHFD2 silencing could potentially impact a number of folate-dependent cytosolic reactions, as well. A similar ‘folate trap’ phenomenon has been observed on loss of cytosolic folate-coupled enzymes, including loss of methionine synthase [33] . Alternatively, loss of MTHFD2 could result in accumulation of a hitherto unknown toxic metabolite that rapidly causes cell death, perhaps from unwanted side reactions of metabolic enzymes occurring in the absence of MTHFD2 (ref. 34 ). While we have consistently observed cell death in response to several independent RNAi sequences targeting MTHFD2 , it must be emphasized that we have hitherto not been able to rescue cell death by overexpression of an RNAi-resistant MTHFD2 cDNA, which is required to conclusively demonstrate that loss of this protein causes cancer cell death. While additional experiments are needed to understand the role of MTHFD2 function in embryonic cells and in cancer, the specific expression of MTHFD2 in transformed cells relative to other adult tissues and the growth and survival defects caused by loss of the mRNA suggests that this enzyme should be evaluated as a potential target for cancer chemotherapeutics. More generally, the current analysis, combined with our previous report [26] and other recent studies [6] , [19] points to a remodelling of mitochondrial one-carbon metabolism in cancer. Although it has long been appreciated that one-carbon folate metabolism is compartmentalized within human cells, these recent studies indicate that compartment-specific alterations may be critical in promoting cancer growth and survival. The recognition that compartmentalization of one-carbon folate metabolism is altered in cancer raises new opportunities for identifying novel therapies for cancer, as well as for targeting existing antifolate therapies with greater precision. Microarray data analysis Microarray data sets were selected from the GCOD [10] according to the following criteria: we considered only data sets of human tumours with normal tissue samples as controls, excluding cell lines and cultured normal cells; we required at least three independent samples in both tumour and control groups; and we considered only data from the Affymetrix HG-Focus, HG-U133A, HG-U133Av2, HG-U133+v2, HG_U95A and HG_U95Av2 microarray platforms. A list of data sets included is provided in Supplementary Data 1 . All data sets were uniformly processed from the Affymetrix CEL using the Robust multi-array average algorithm, as described [10] . For each microarray platform, in cases of multiple probe sets per gene, we selected the probe set with a maximal mean signal rank across all arrays. Differential expression between tumour and normal groups was quantified for each data set using Z -scores, and nominal P -values of differential expression were calculated for each gene using a permutation test (1,000 permutations). FDRs were computed using the Benjamini–Hochberg procedure [35] . Meta-analysis of the FDR was done by counting the number of times a gene was overexpressed in tumours and subtracting the number of times it was underexpressed. Enrichment analysis was done using the GSEA-p method [36] with the parameter p set to 1. The compendium of 80 human tissues was generated from duplicate samples for each tissue using Affymetrix U133A arrays [37] . The gcRMA-normalized data was downloaded from www.biogps.org , and duplicates were averaged for the analysis presented in Fig. 2 . Our classification of tissues and cells as normal/postmitotic, normal/proliferating or transformed is described in Supplementary Table 1 . Expression data from proliferating human fibroblasts, human T cells, mouse regenerating liver and mouse/human embryonic development was obtained from the NCBI Gene Expression Omnibus, series accession GSE3945 , GSE2770 , GSE6998 and GSE18290 , respectively. No additional normalization was performed. Cell culture Human cancer cell lines (passage number 5–18 in all cases except HCT-116) were obtained from the National Cancer Institute. All cell lines were cultured in RPMI-1640 medium (Invitrogen) with 2 mM L -glutamine and 5% fetal bovine serum (FBS) (HyClone Laboratories). Cells were cultured at 37 °C in 5% CO 2 . shRNA knockdown of MTHFD2 Cells were cultured according to standard techniques as described above. Lentiviral vectors (pLKO.1) expressing shRNA clones were generated by the Broad RNAi Consortium, as previously described [26] . Sequence-independent shRNAs were generated against human MTHFD2 (sh50, sh53) or a control sequence (shCtrl) not matching any human gene. Accession numbers are: shCtrl, Clone ID TRCN0000072232, Clone name lacZ_27s1c1, Target sequence 5′-CGTCGTATTACAACGTCGTGA-3′; shD2-50, Clone ID TRCN0000036550, Clone name NM_006636.2-548s1c1, Target sequence 5′-CGAATGTGTTTGGATCAGTAT-3′; shD2-53, Clone ID TRCN0000036553, Clone name NM_006636.2-772s1c1, Target sequence 5′-GCAGTTGAAGAAACATACAAT-3′. The pLKO.1 plasmids were each packaged with VSVG and pCMV-dR8.91 vectors in 293T cells to generate lentivirus, as previously described [26] . One day before transfection, 850,000 293T cells were seeded per well/plasmid. Roche X-tremeGENE 9 was used to transfect 293T cells according to the manufacturer's protocols (100 ng VSVG, 900 ng pCMV-dR8.91 and 1 μg plasmid with 6 μl transfection reagent for each well/plasmid). After 18 h of transfection, high serum (30% Gibco 16,000 FBS in DMEM) media was added. Virus was harvested at 24 and 48 h, pooled and frozen at −80C in single-use aliquots [26] . Lentiviral infection was performed as previously described [26] . Cells were seeded at a density of 1,500–2,500 cells per well, depending on cell type, in a 96-well plate in RPMI-1640 medium (200 μl total) supplemented with 5% FBS and 2 mM glutamine. Fifteen hours after plating, the cell culture medium was exchanged with fresh medium containing polybrene (8 μg ml −1 ) and viral supernatant. Plates were centrifuged for 30 min at 2,000 g and 37 °C, after which the medium was replaced. Twenty-four hours later, cells were selected for infection by adding puromycin to the cell culture medium (2 μg ml −1 ). Uninfected control cells demonstrated 100% cell death within 48 h. Seven days following plating, cells were washed with phosphate-buffered saline and fixed using 4% paraformaldehyde for 20 min at room temperature. Cells were stained using the Hoechst 33,342 dye (Invitrogen) according to manufacturer’s specifications, imaged using an ImageXpress Micro (Molecular Devices), and counted using the ‘count nuclei’ module of MetaXpress (Molecular Devices). Cell counts are expressed normalized to shCtrl-infected cells for each cell line. All experiments were performed using at least four independent cell cultures. For MTHFD2 mRNA and protein measurements following shRNA knockdown, HCT-116 cells were infected with lentiviral shRNA vectors in six-well dishes as described [26] . Seven days following infection, mRNA was isolated from cells using an RNeasy kit (Qiagen), and quantitative reverse transcription-PCR was performed for MTHFD2 and HPRT using the Taqman assays (Applied Biosystems, assay ID Hs01074341_g1 and Hs99999909_m1, respectively), according to the manufacturer’s instructions. Quantitative reverse transcription-PCR data are expressed as ΔΔ C T values. For western blot analysis, whole-cell lysates were prepared and resolved by SDS–PAGE, followed by transfer to a PVDF membrane using the Trans-Blot Turbo Transfer System. Membranes were stained using primary antibody for ATP5A (Abcam mouse monoclonal, no. AB147480, 1:100,000) or MTHFD2 (Abcam mouse monoclonal, no. AB56772, 1:500), followed by secondary antibody (polyclonal sheep anti-IgG mouse antibody, no. NA931V, 1:10,000). The signal was detected using enhanced chemiluminescence. Full images of western blots are provided in Supplementary Fig. 3a . For assay of MTHFD2 activity, 1 × 10 6 cells were lysed in 24% glycerol, 1% Triton-X diluted in phosphate-buffered saline (pH 7.4) and MTHFD2 activity measured in lysate, as previously described [28] . Transient siRNA knockdown siRNA oligonucleotides targeting MTHFD2 were from Dharmacon, catalogue no. J-009349-10, J-009349-11, J-009349-12, D-009349-02, D-0093848-03 and D-009349-04, referred to in this study as siD2-10, siD2-11, siD2-12, siD2-2, siD2-3 and siD2-3, respectively. Control siRNAs were Dharmacon ON-TARGET, referred to as siCtrl-1, and Dharmacon siGenome, referred to as siCtrl-2. Cells were transfected 24 h after seeding (at 40–60% confluence) with 10 nM oligonucleotide, using the INTERFERin transfection reagent (Polyplus Transfection). Western blot analysis was performed on cells seeded at 150,000 cells per well in a six-well plate and lysed in 2 × Laemmli sample loading buffer 48 h after siRNA transfection. Lysates were separated by 10% Mini-PROTEAN TGX Precast Gel (Bio-Rad), transferred to a 0.45-μm nitrocellulose membrane (Bio-Rad) and blocked in 5% milk in tris-buffered saline and Tween-20. The following antibodies were used for immunoblotting: monoclonal mouse β-actin antibody (Sigma-Aldrich, 1:30,000), monoclonal mouse MTHFD2 (Abnova, no. H00010797-M01, 1:500) and anti-mouse IgG (H+L) HRP conjugated (Pierce, 1:100,000). Full images of western blots are provided in Supplementary Fig. 3b . For assessment of cellular proliferation following transient siRNA transfection, cells were seeded at 4,000 cells per well in a 96-well plate 24 h before siRNA transfections and lysed at the indicated time points using the CyQuant Cell Proliferation Assay (Invitrogen) according to manufacturer’s instructions. Binding of CyQuant to DNA was analysed by measuring fluorescence in a VICTOR2 plate reader (PerkinElmer). Flow cytometric measurement of cell death Cells were seeded at 10 6 cells per 100 mm dish 24 h before siRNA transfections. Cells were collected by trypsinization at the indicated time points, pelleted for 5 min at 1,500 g , rinsed twice in ice-cold phosphate-buffered saline and then resuspended in 0.01 M HEPES/NaOH (pH 7.4), 0.14 M NaCl and 2.5 mM CaCl 2 . The cell suspension was diluted to a concentration of 5 × 10 5 cells ml −1 , 2.5 × 10 5 cells were transferred to a 5-ml culture tube and PI(BD Pharmingen) was added at a concentration of 0.5 μg ml −1 ; cells were gently vortexed and incubated for 15 min at 25 °C in the dark. Samples were analysed within 1 h in a CyAn ADP Analyzer (Beckamn Coulter), with a flow rate ~300 events s −1 and a total of 25,000 events were gated. Debris and doublets were excluded using forward scatter and pulse width before gating of PI-positive populations. Immunohistochemistry Specimens containing normal and/or cancer tissues were collected in accordance with approval from the local ethics committee (ref no. Ups 02–577) and according to Swedish rules and legislation. Tissue microarrays holding samples from the different cancer types as well as from normal tissues were produced, as previously described [38] . Briefly, tissue samples were fixed with formalin and embedded in paraffin; 2–3 tissue cylinders from representative areas were punched out and assembled in a recipient tissue microarray block with prepunched holes. For immunohistochemical staining 4 μm sections were then cut and placed on Superfrost Plus microscope slides (Thermo Fisher Scientific, Fremont, CA, USA). Slides were deparaffinized in xylene, hydrated in graded alcohols and blocked for endogenous peroxidase for 5 min in 0.3% H 2 O 2 diluted in 95% ethanol. Heat-induced epitope retrieval was done in a decloaking chamber (Biocare Medical) with citrate buffer at pH 6.0 for 4 min at 125 °C. Before staining, slides were immersed in wash buffer containing 0.2% Tween-20 for 15 min to avoid surface tension. Staining was performed in an Autostainer 480S instrument (Thermo Fisher Scientific) at room temperature with the following steps: Ultra V block (Thermo Fisher Scientific, no. TA-125-UB) 5 min, primary antibody 30 min, primary antibody enhancer (Thermo Fisher Scientific, no. TL-125-PB) 20 min, UltraVision LP HRP polymer (Thermo Fisher Scientific, no. TL-125-PH) 30 min and diaminobenzidine (Thermo Fisher Scientific, no. TA-125-HDX) 5 min two times. MTHFD2 primary antibody was from Abnova (mouse monoclonal, no. H00010797-M01). Between incubations, slides were rinsed in wash buffer. Slides were counter-stained with Mayer’s hematoxylin (Histolab, Gothenburg, Sweden, ref. 01820), dehydrated and mounted on cover slips using pertex (Histolab, ref. 00871.0500). Two independent observers evaluated staining for all samples, blinded to the identity of the antibodies used. Staining intensity was classified (negative, weak, moderate and strong) and fraction of positive cells (0, <25%, 25–75%, >75%) were estimated separately for tumour cells and tumour stroma. Survival analysis Six independent large cohorts of cancer patients for which survival data for at least a decade were available were examined. Microarray data from Chin et al. [39] and van de Vijver et al. [40] , were downloaded from the Lawrence Berkeley National Laboratory ( http://cancer.lbl.gov/breastcancer/list_data.php?id=9 ) and Rosetta Inpharmatics ( http://www.rii.com/publications/2002/nejm.html ), respectively. Microarray data from the Desmedt et al. [41] , Pawitan et al. [42] , Miller et al. [43] and Kao et al. [44] studies are available from the NCBI Gene Expression Omnibus, accessions GSE7390 , GSE1456 , GSE3494 and GSE20685 , respectively. Survival data and clinical parameters were obtained from the original reports. Patients were split into ‘positive’ or ‘negative’ based on above- or below-median expression of the MTHFD2 mRNA, and Kaplan–Meier curves were derived for these groups. Hazard ratios were estimated using Cox's proportional hazard model [45] . Groups were tested for significant differences using the logrank test, and meta-analysis was performed using the method by DerSimonian and Laird [46] . How to cite this article: Nilsson, R. et al. Metabolic enzyme expression highlights a key role for MTHFD2 and the mitochondrial folate pathway in cancer. Nat. Commun. 5:3128 doi: 10.1038/ncomms4128 (2014).